Origin of synergistic effects in bicomponent cobalt oxide-platinum catalysts for selective hydrogenation reaction The synergistic nature of bicomponent catalysts remains a challenging issue, due to the difficulty in constructing well-defined catalytic systems. Here we study the origin of synergistic effects in CoO x -Pt catalysts for selective hydrogenation by designing a series of closely contacted CoO x Pt/TiO 2 and spatially separated CoO x /TiO 2 /Pt catalysts by atomic layer deposition (ALD). For CoO x /TiO 2 /Pt, CoO x and platinum are separated by the walls of titania nanotubes, and the CoO x -Pt intimacy can be precisely tuned. Like CoO x Pt/TiO 2 , the CoO x /TiO 2 /Pt shows higher selectivity to cinnamyl alcohol than monometallic TiO 2 /Pt, indicating that the CoO x -Pt nanoscale intimacy almost has no influence on the selectivity. The enhanced selectivity is ascribed to the increased oxygen vacancy resulting from the promoted hydrogen spillover. Moreover, platinum-oxygen vacancy interfacial sites are identified as the active sites by selectively covering CoO x or platinum by ALD. Our study provides a guide for the understanding of synergistic nature in bicomponent and bifunctional catalysts. Bicomponent catalysts have received considerably increasing interests in the recent decades due to the enhanced catalytic properties compared with their single-component counterparts, arising from direct contact between the two components, which can be called as synergistic effects [1] , [2] . However, due to the limitations in controlling the catalyst microstructures and precisely tuning bicomponent intimacy by the traditional methods, it is still a challenging issue to understand the origin of synergistic effects (i.e., short- or long-range interactions) and identify the active sites. The general belief is that the bicomponents should be as close as possible (i.e., short-range interactions of bicomponents) to promote electron interaction and/or construct interfaces to achieve effective catalysis. In this case, the interaction of a metal oxide promoter with a metal particle is puzzling due to the presence of multiple potential catalytic active sites under the reaction conditions. In contrast, some recent reports revealed the effects of intimacy on the catalyst performance when the bicomponents are separated and tuned at nanoscale and even millimeter-scale distance (i.e., long-range interactions of bicomponents) [3] , [4] , [5] , [6] , [7] , [8] , [9] , [10] . For example, Coville and coworkers investigated the effect of Ru and Co intimacy on the activity and selectivity of Co catalysts using conventional incipient wetness impregnation in the typical Fischer–Tropsch reaction [5] . Bokhoven and coworkers prepared a series of model catalyst samples with precisely controlled Pt–FeO x intimacy at nanoscale distances using the more precise nanolithography technique, and investigated the hydrogen spillover effects on TiO 2 and Al 2 O 3 supports [7] . But no reaction (not possible for such structure) is conducted to verify the proposed hydrogen spillover mechanism under the real reaction conditions. Therefore, well-defined bicomponent catalytic systems are highly desirable to unravel the origin of synergistic effects under the real reaction conditions. Atomic layer deposition (ALD) is a powerful thin-film technique for synthesis of conformal thin films and highly dispersed nanoparticles [11] , [12] , [13] , [14] , [15] , [16] . Many advanced nanocatalysts have been designed and synthesized by ALD in the past decade [17] , [18] , [19] , [20] , [21] , [22] , [23] , [24] , [25] , [26] . Herein, we investigate the effects of CoO x –Pt intimacy on the selective hydrogenation of cinnamaldehyde (CALD) and the hydrogen spillover effects based on CoO x Pt/TiO 2 and well-designed spatially separated structures of CoO x /TiO 2 /Pt catalysts by a highly controllable and reliable ALD approach. Compared with the CoO x Pt/TiO 2 , the CoO x /TiO 2 /Pt catalysts exhibit similar catalytic activity and hydrogenation selectivity for the CALD hydrogenation, though the CoO x –Pt intimacy of the two catalysts is dramatically different. This long-range promoter effect is not broken even when we selectively deposit additional coating layers on the CoO x surfaces by ALD. The enhanced selectivity is ascribed to the promoted hydrogen spillover and thus increased oxygen vacancies (O v ). The well-designed structures can be synthesized and used to study the synergetic natures of other bicomponent and bifunctional catalysts with enhanced performance for other reactions. Synthesis and characterization of the catalysts The closely contacted CoO x Pt/TiO 2 and spatially separated CoO x /TiO 2 /Pt catalysts were synthesized by a template-assisted ALD strategy (Fig. 1 and Supplementary Scheme 1 ) [26] . For the synthesis of CoO x Pt/TiO 2 , an amorphous TiO 2 film was first deposited on carbon nanocoils (CNCs) used as templates by ALD, obtaining TiO 2 /CNCs, and then Pt nanoparticles were deposited on the TiO 2 /CNCs by Pt ALD, obtaining Pt/TiO 2 /CNCs. Subsequently, the CNCs were removed by calcination under an air atmosphere, producing Pt/TiO 2 catalysts with anatase nanotubes. Lastly, CoO x nanoparticles were deposited on the outer surface of the Pt/TiO 2 through CoO x ALD, producing CoO x Pt/TiO 2 catalysts with the closest CoO x –Pt intimacy (Supplementary Scheme 1a ). The CoO x /TiO 2 /Pt catalysts were prepared by exchanging the deposition sequence of TiO 2 and Pt (Supplementary Scheme 1b ). The CoO x –Pt intimacy can be precisely controlled by adjusting the thickness of TiO 2 layer. In addition, the CoO x /TiO 2 /Pt/TiO 2 and Al 2 O 3 /CoO x /TiO 2 /Pt catalysts (Fig. 1 ) were also prepared by selectively covering Pt with TiO 2 and CoO x nanoparticles with Al 2 O 3 , respectively, to identify the real active sites in the bicomponent catalysts. Fig. 1 Schematic illustration of the catalysts. Semi-sectional and cross-sectional views of the different catalysts prepared by ALD. The yellow and black balls represent Pt and CoO x , respectively Full size image Figure 2 shows the transmission electron microscopy (TEM) and high-resolution TEM (HRTEM) images of the CoO x Pt/TiO 2 and CoO x /TiO 2 /Pt catalysts, prepared with 150, 20 and 300 cycles for CoO x , Pt and TiO 2 deposition, respectively. 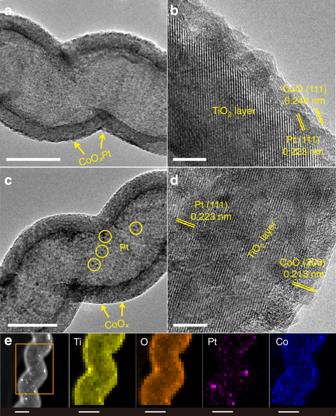Fig. 2 Structural characterizations of the two catalysts. TEM and HRTEM images of the CoOxPt/TiO2(a,b) and CoOx/TiO2/Pt (c,d) catalysts.eSTEM image of the CoOx/TiO2/Pt catalysts and the corresponding EDS mapping profiles in rectangular area. Scale bars:a,cande50 nm;bandd5 nm The Pt and CoO x nanoparticles, with average sizes of 2.9 nm and 4.3 nm, respectively (Supplementary Figs. 1 and 2 ), are highly dispersed on the outer surface of the anatase TiO 2 nanotubes with a wall thickness of ~13.7 nm, in which CoO x is deposited on/next to Pt forming CoO x –Pt interfaces (Fig. 2a, b ). The measured lattice distances of the nanoparticles are ~0.223 nm and ~0.246 nm (Fig. 2b ), which correspond to the Pt(111) and CoO (111) planes, respectively [27] , [28] . The larger lattice distance of 0.350 nm matches well with (101) planes of anatase TiO 2 [26] . For the CoO x /TiO 2 /Pt catalyst (Fig. 2c, d ), Pt nanoparticles (indicated by yellow circles) with an average particle size of 3.1 nm (Supplementary Fig. 3 ) are uniformly deposited on the inner surface of the TiO 2 nanotubes, while CoO x nanoparticles are uniformly deposited on the outer surface of the TiO 2 nanotubes (Supplementary Fig. 4 ). In CoO x Pt/TiO 2 catalysts, the Pt nanoparticles are closely contacted with CoO x nanoparticles, while in CoO x /TiO 2 /Pt catalysts, the average CoO x –Pt distance is corresponded to the TiO 2 thickness. Thus the average CoO x –Pt distance in CoO x Pt/TiO 2 is much smaller than that of CoO x /TiO 2 /Pt. The sample was further characterized by using high-angle annular dark-field scanning TEM (HAADF-STEM), and energy-dispersive X-ray spectroscopy (EDS) mapping (Fig. 2e and Supplementary Figs. 5 and 6 ), further confirming that the Pt and CoO x nanoparticles are separately decorated on the inner and outer surfaces of the TiO 2 nanotubes, respectively. Fig. 2 Structural characterizations of the two catalysts. TEM and HRTEM images of the CoO x Pt/TiO 2 ( a , b ) and CoO x /TiO 2 /Pt ( c , d ) catalysts. e STEM image of the CoO x /TiO 2 /Pt catalysts and the corresponding EDS mapping profiles in rectangular area. Scale bars: a , c and e 50 nm; b and d 5 nm Full size image Catalytic performance The selective hydrogenation of C=O in α, β-unsaturated aldehydes (e.g., CALD) to value-added unsaturated alcohols has been of increasing interest for the production of fine chemicals and pharmaceutical precursors [29] , [30] , [31] , [32] , [33] , [34] , [35] , [36] , [37] , [38] . However, it remains challenging to achieve high-yield unsaturated alcohols since the hydrogenation of C=C is thermodynamically more favorable than that of C=O. To address the issue, various catalysts have been designed and synthesized, and Pt-based catalysts were found to be more desirable in the selective reduction of C=O than other metals [29] , [30] , [31] , [32] , [33] , [34] , [35] , [36] , [37] , [38] . Bitter and coworkers found that Pt particle size and oxygen groups on carbon nanofiber supports have a vital influence on the selectivity to cinnamyl alcohol (CALC) [29] . Chen and coworkers reported that Co–Pt/SiO 2 bimetallic catalysts exhibit better catalytic activity and selectivity than Pt/SiO 2 and Cu–Pt/SiO 2 catalysts due to the electronic property modification of Pt [30] , [31] . 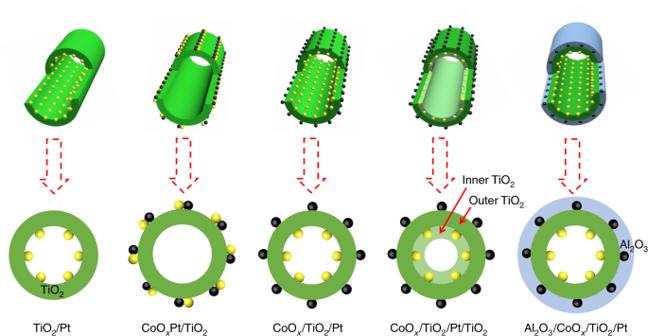Similar results were also reported by Tsang et al., i.e., the selective C=O hydrogenation can be achieved with high activity using Co-decorated Pt nanocrystals as nanocatalysts [38] . Fig. 1 Schematic illustration of the catalysts. Semi-sectional and cross-sectional views of the different catalysts prepared by ALD. The yellow and black balls represent Pt and CoOx, respectively To unravel the synergetic mechanism, the selective hydrogenation of CALD is selected as an example to evaluate the catalytic properties of the as-prepared catalysts, and the results are summarized in Table 1 . Note that the Pt nanoparticles are located at different positions for the Pt/TiO 2 and TiO 2 /Pt catalysts. For the monometallic TiO 2 /Pt catalyst with Pt loading of 3.7 wt.% (Supplementary Table 1 ), the main product is hydrocinnamaldehyde (HALD) obtained from hydrogenation of the C=C and the selectivity to HALD amounts to 62.5%, while the selectivity to the desired product CALC, obtained from hydrogenation of the C=O, is only 16.2% (Entry 1). For the CoO x /TiO 2 reference catalyst, only trace conversion (0.9%) is detected under the same reaction conditions (Entry 2). For the CoO x Pt/TiO 2 catalysts with closely contacted Pt and CoO x , the selectivity to CALC is remarkably improved after addition of CoO x (Entry 3). Moreover, the product of excessive hydrogenation to hydrocinnamyl alcohol (HALC) is also obviously suppressed. Similar phenomenon is also found for the CoO x -supported Pt-based catalysts, and the Pt40/CoO x catalysts exhibit the best catalytic performance with 90.2% conversion and 80.3% selectivity to CALC (Supplementary Fig. 7 ). The improved selectivity to CALC is usually ascribed to the promoter effects, originating from electronic or structural modifications [35] , [36] , [37] , [38] , [39] , [40] , [41] . Unexpectedly, similar hydrogenation results are also achieved over the CoO x /TiO 2 /Pt (13.7 nm, 300-cycle TiO 2 ) catalysts with nanoscale CoO x –Pt intimacy (Entry 4 and Supplementary Fig. 8 ). Moreover, only slight decrease in hydrogenation activity and selectivity is observed over the CoO x /TiO 2 (900)/Pt catalysts (Entry 5) when the TiO 2 layer becomes much thicker (40.5 nm, 900-cycle TiO 2 , Supplementary Figs. 9 and 10 ). Table 1 Selective hydrogenation results of CALD over the different catalysts a Full size table Furthermore, control experiments were also carried out by selectively exposing Pt or CoO x to confirm the roles played by CoO x and Pt during the reaction. The hydrogenation conversion and selectivity to the desired CALC product decrease remarkably when Pt is selectively covered by two-layered TiO 2 (CoO x /TiO 2 /Pt/TiO 2 , Entry 6). When CoO x is selectively covered by an outer dense Al 2 O 3 layer of ~11.5 nm (Al 2 O 3 /CoO x /TiO 2 /Pt), no visible change is observed in the catalytic performance (Entry 7). These results indicate that Pt–TiO 2 interface regions should be the main active sites for the CALD hydrogenation reaction, instead of CoO x . It should be noted that the selectivity of CALC hydrogenation is guaranteed to improve with CoO x addition due to the long-range promoter effect and that this effect is not broken even when the surface of CoO x promoter is entirely covered by a dense Al 2 O 3 layer (Al 2 O 3 /CoO x /TiO 2 /Pt, Entry 7). This effect is altered when the TiO 2 layer is changed to Al 2 O 3 (~11.5 nm), i.e., the catalytic performance is considerably influenced by the CoO x –Pt intimacy (Entries 8–11). Closely contacted CoO x Pt/Al 2 O 3 catalysts exhibit higher activity and selectivity to the desired product than those of the separated CoO x /Al 2 O 3 /Pt catalysts with nanoscale intimacy. This should be related to the poor capability of spillover hydrogen transfer on the nonreducible Al 2 O 3 [7] . In addition, the reusability of CoO x /TiO 2 /Pt for selective hydrogenation of CALD was also tested (Supplementary Fig. 11 ). There is no obvious decrease in the conversion after five catalytic cycles, indicating a good stability of the catalysts. X-ray absorption fine structure measurements The electronic states of the TiO 2 /Pt, CoO x /TiO 2 /Pt and CoO x Pt/TiO 2 catalysts before and during the hydrogenation reaction processes were investigated by ex situ and in situ X-ray absorption fine structure measurements (Fig. 3 ). 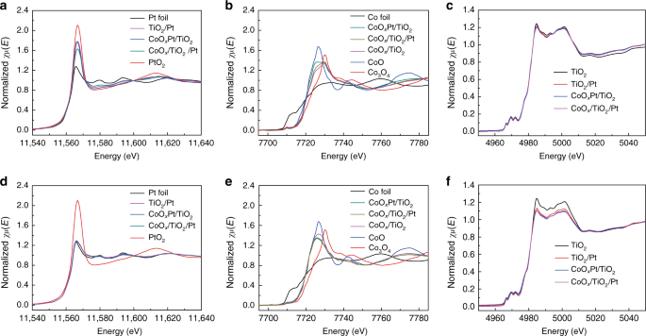Fig. 3 XANES spectra of the catalysts.aEx situ anddin situ Pt L3-edge XANES spectra of TiO2/Pt, CoOx/TiO2/Pt, CoOxPt/TiO2, and reference Pt foil and PtO2;bEx situ andein situ Co K-edge XANES spectra of TiO2/Pt, CoOx/TiO2/Pt, CoOxPt/TiO2, and reference Co foil, CoO and Co3O4;cEx situ andfin situ Ti K-edge XANES spectra of TiO2/Pt, CoOxPt/TiO2, CoOx/TiO2/Pt and reference TiO2 Figure 3a shows the normalized Pt L 3 -edge ex situ X-ray absorption near-edge structure (XANES) spectra of the as-prepared catalysts, and the reference spectra of Pt foil and PtO 2 . The white line intensity of the as-prepared catalysts falls in the range between the Pt foil and PtO 2 , suggesting that the as-prepared Pt nanoparticles consist of a certain amount of PtO x in addition to metallic Pt 0 . Expanded view of the white lines (Supplementary Fig. 12 ) indicates the different electronic states of Pt for TiO 2 /Pt, CoO x /TiO 2 /Pt and CoO x Pt/TiO 2 catalysts. Figure 3b presents the normalized Co K-edge XANES spectra of the as-prepared catalysts before the reaction, and the reference spectra of Co foil, CoO and Co 3 O 4 . Obviously, the CoO x /TiO 2 /Pt catalysts also exhibit different white line shapes in comparison with the CoO x Pt/TiO 2 catalysts, indicating the different electronic states of the CoO x species between the two catalysts. These results demonstrate that before the reaction, the electronic interaction between CoO x promoter and Pt should exist (Supplementary Fig. 13 ). During the reaction process, the PtO x species of TiO 2 /Pt, CoO x /TiO 2 /Pt and CoO x Pt/TiO 2 are fully reduced to metallic Pt 0 due to the presence of H 2 (Fig. 3d ). The Fourier transform spectra of the Pt L 3 -edge extended X-ray absorption fine structure (EXAFS) oscillations for these three catalysts also confirm the full reduction of PtO x during the reaction process (Supplementary Fig. 14a, b ). For the CoO x /TiO 2 reference catalysts, the white line shifts to a low energy during the reaction process (Fig. 3b and e), indicating that the cobalt oxide species at high valence could be reduced to relatively low valence states (e.g., from Co 3 O 4 to CoO) under a H 2 atmosphere without Pt assistance (Supplementary Fig. 14c, d ). Lower energy shifts of the white lines can be observed for the CoO x Pt/TiO 2 and CoO x /TiO 2 /Pt catalysts during the reaction process, demonstrating that more cobalt oxide species with lower valence states are formed in the two catalysts compared with the CoO x /TiO 2 catalysts, which can be ascribed to the presence of Pt contributing to the reduction of CoO x due to the hydrogen spillover effect. In addition, the CoO x Pt/TiO 2 and CoO x /TiO 2 /Pt catalysts exhibit almost the same white line shapes during the reaction process (Fig. 3e ), i.e., the valence states of the formed cobalt oxide species of the two catalysts are nearly identical; this is due to the strong reduction ability of the spillover hydrogen (H·), generated on Pt, toward CoO x , which is nearly independent of the CoO x –Pt intimacy on reducible TiO 2 supports in the nanoscale range [7] . Fig. 3 XANES spectra of the catalysts. a Ex situ and d in situ Pt L 3 -edge XANES spectra of TiO 2 /Pt, CoO x /TiO 2 /Pt, CoO x Pt/TiO 2 , and reference Pt foil and PtO 2 ; b Ex situ and e in situ Co K-edge XANES spectra of TiO 2 /Pt, CoO x /TiO 2 /Pt, CoO x Pt/TiO 2 , and reference Co foil, CoO and Co 3 O 4 ; c Ex situ and f in situ Ti K-edge XANES spectra of TiO 2 /Pt, CoO x Pt/TiO 2 , CoO x /TiO 2 /Pt and reference TiO 2 Full size image Figure 3c and f shows the normalized Ti K-edge ex situ and in situ XANES spectra of TiO 2 /Pt, CoO x /TiO 2 /Pt, CoO x Pt/TiO 2 and the reference spectra of TiO 2 . Before the reaction, the Ti K-edge white line curves of all the three catalysts coincide, indicating the same electronic states of their TiO 2 supports. During the hydrogenation reaction conditions, in situ XANES spectra show reduction of Ti 4+ to Ti 3+ for all three catalysts, and CoO x /TiO 2 /Pt and CoO x Pt/TiO 2 possess more reduced Ti 3+ than that of the TiO 2 /Pt catalyst. The k 3 -weighted EXAFS spectra of the three catalysts and the reference TiO 2 , and their fitted curves are presented in Supplementary Fig. 15 . The fitted results (Supplementary Table 2 ) are consistent with the XANES results. 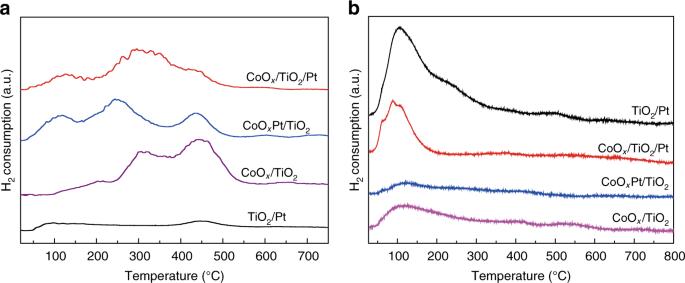Fig. 4 Chemisorption characterizations.aH2-TPR andbH2-TPD profiles of the catalysts 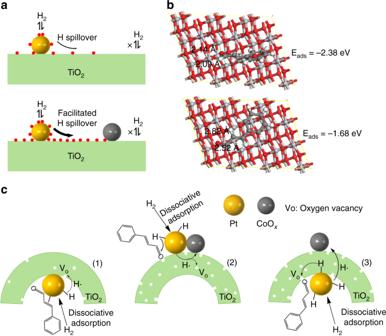Fig. 5 DFT calculation and proposed reaction mechanisms.aThe effect mechanism of CoOxon the hydrogen spillover over TiO2-supported Pt catalysts.bThe optimized structure for adsorption of CALD molecule using C=O (top) or C=C (bottom) double bond on the Ovof TiO2. Atom coloring: Ti, gray; O, red; H, white; C, black.cThe possible enhancement mechanism for selective CALD hydrogenation reaction. (1), (2) and (3) represent TiO2/Pt, CoOxPt/TiO2and CoOx/TiO2/Pt catalysts, respectively. For TiO2/Pt, the number of Ovis limited, leading to its low selectivity. For CoOxPt/TiO2and CoOx/TiO2/Pt, the addition of CoOxpromotes the formation of Ovsites through hydrogen spillover and thus improves the selectivity, regardless of whether CoOxand Pt are separated by a TiO2layer or not Chemisorption Figure 4a shows the H 2 temperature programmed reduction (H 2 -TPR) profiles of the catalysts. From the H 2 -TPR profiles of the CoO x Pt/TiO 2 , CoO x /TiO 2 /Pt and CoO x /TiO 2 catalysts (also see Supplementary Fig. 10 ), both a low temperature (110–220 °C, Co 3 O 4 to CoO) and a high temperature (245–345 °C, CoO to Co 0 ) reduction peak can be observed. No peaks related to platinum oxides are observed, probably because the amounts of H 2 used for the reduction of PtO x species in the catalysts are beyond the lower detection limits of the detector. In addition, the reduction peak at higher temperature (~450 °C) could be assigned to the partial reduction of TiO 2 , indicating that TiO 2 is more difficult to reduce [42] . Compared with the CoO x /TiO 2 catalysts, the temperatures needed for CoO x reduction are much lower for the CoO x Pt/TiO 2 and CoO x /TiO 2 /Pt catalysts due to the presence of Pt, further revealing the effect of hydrogen spillover from Pt to CoO x [31] . Note that the reduction temperature needed for the CoO x Pt/TiO 2 catalyst is slightly lower than that of the CoO x /TiO 2 /Pt catalyst due to the closer CoO x –Pt intimacy (Fig. 4a ). Figure 4b shows the H 2 temperature programmed desorption (H 2 -TPD) profiles of the catalysts. The TiO 2 /Pt and CoO x /TiO 2 /Pt catalysts exhibit a much higher H 2 adsorption ability than that of the CoO x /TiO 2 and CoO x Pt/TiO 2 catalysts, indicating that Pt atoms are the adsorption and dissociation sites of H 2 , which is further verified by the following density functional theory (DFT) simulation. Fig. 4 Chemisorption characterizations. a H 2 -TPR and b H 2 -TPD profiles of the catalysts Full size image In this work, we discovered a hydrogen spillover effect for the CALD hydrogenation reactions. Hydrogen spillover is a reversible and dynamic equilibrium process. Modulation of the spillover conditions, such as temperature and gas partial pressure, hinders or facilitates the spillover process and can be used for controlling the oxide reduction [7] , [43] . Generally, the activation and dissociation of H 2 molecules on Pt is quite easy and generally considered to be barrierless [7] , [43] , [44] , [45] , i.e., the energy needed to activate H 2 molecules on Pt is much lower than that on CoO x and TiO 2 (Supplementary Fig. 16 ). For the TiO 2 /Pt catalyst under the reaction conditions, hydrogen spillover occurs (Fig. 5a ). Active hydrogen species migrate from Pt onto TiO 2 supports, leading to the partial reduction of TiO 2 supports (Ti 4+ is reduced to Ti 3+ ) with the formation of O v around the interface regions [7] , [46] , [47] , [48] , [49] , [50] . When CoO x is added, in situ XAFS results show that CoO x can be reduced to lower valent states through hydrogen spillover under the reaction conditions. More hydrogen species are consumed by CoO x , thus the original equilibrium of hydrogen spillover is disturbed (Fig. 5a ). The generation of active hydrogen species and their transfer process (from Pt to CoO x directly, or via TiO 2 supports) are promoted, until new equilibrium is reached. The consumption of hydrogen species can be seen as the pumps for the migration of atomic hydrogen from Pt toward TiO 2 . The enhanced hydrogen spillover facilitates the reduction of TiO 2 supports, which is proved by in situ Ti K-edge XANES spectra (Fig. 3c and f), accompanying the increased formation of O v sites. Fig. 5 DFT calculation and proposed reaction mechanisms. a The effect mechanism of CoO x on the hydrogen spillover over TiO 2 -supported Pt catalysts. b The optimized structure for adsorption of CALD molecule using C=O (top) or C=C (bottom) double bond on the O v of TiO 2 . Atom coloring: Ti, gray; O, red; H, white; C, black. c The possible enhancement mechanism for selective CALD hydrogenation reaction. (1), (2) and (3) represent TiO 2 /Pt, CoO x Pt/TiO 2 and CoO x /TiO 2 /Pt catalysts, respectively. For TiO 2 /Pt, the number of O v is limited, leading to its low selectivity. For CoO x Pt/TiO 2 and CoO x /TiO 2 /Pt, the addition of CoO x promotes the formation of O v sites through hydrogen spillover and thus improves the selectivity, regardless of whether CoO x and Pt are separated by a TiO 2 layer or not Full size image The adsorption energies of different adsorption configurations of a CALD molecule on the O v formed on TiO 2 were calculated (Fig. 5b ). The calculated adsorption energy of the C=O bond adsorbed on the oxygen vacancies is −2.38 eV, which is larger than that of the C=C bond on the oxygen vacancies (−1.68 eV), indicating that the adsorption configurations of the CALD molecule through the C=O bond on the O v are more stable. Based on the above discussions, the possible enhancement mechanism is proposed. For the TiO 2 /Pt catalyst, the number of O v at the Pt–TiO 2 interface is limited under the reaction conditions, leading to its low selectivity (Fig. 5c ). When CoO x promoters are added, the selectivity to CALC is improved. The promotion can be ascribed to the CoO x promoter-induced increase of O v sites through hydrogen spillover effect. For CoO x /TiO 2 /Pt catalysts, although CoO x is separated from the Pt catalyst by a TiO 2 layer, this long-range CoO x promoter can still enhance the catalytic selectivity to CALC. XAFS results demonstrate that the electronic states of CoO x of CoO x Pt/TiO 2 and CoO x /TiO 2 /Pt catalysts are almost the same during the reaction process, meaning that the active hydrogen species generated on Pt nanoparticles are still consumed by CoO x , though CoO x is far from Pt. The energy barrier for the transfer of an electron and a proton among the different TiO 2 sites can be easily overcome under the reaction conditions [7] , and thus the distance of hydrogen spillover across TiO 2 layer almost has no influence on the catalytic performance. The addition of CoO x results in the increased generation of O v sites on the Pt–TiO 2 interface regions and the remarkably improved selectivity to CALC. To further clarify the long-range promoter effect (i.e., the role of CoO x played), we selectively deposit additional oxide layers on the surfaces of CoO x or Pt by ALD. From the XAFS results, it can be concluded that CoO x species in the catalysts can be reduced in two ways. Firstly, the CoO x species can be reduced under H 2 atmosphere; secondly, the CoO x species can be further reduced to a lower valence state by the active H species spilled from Pt nanoparticles through TiO 2 support. When Pt is selectively covered by TiO 2 (CoO x /TiO 2 /Pt/TiO 2 ), the access of CALD molecules to Pt is nearly blocked due to the diffusion limitation (Supplementary Figs. 17 and 18 , Supplementary Table 3 ), leading to the decreased catalytic performance (Entry 6, Table 1 ). On the contrary, when CoO x is selectively covered by a dense Al 2 O 3 layer (Al 2 O 3 /CoO x /TiO 2 /Pt), the first way is blocked (Supplementary Fig. 18 ), while the second way is still preserved and CALD molecules can still have access to Pt via open the ends of the TiO 2 nanotubes (with a diameter of ~70–90 nm), leading to a nearly unchanged catalytic performance (Entry 7, Table 1 ). These results further demonstrate that H spillover way is the main path to improve selectivity, and that Pt–O v interface instead of CoO x should be the active site for the CALD hydrogenation reaction. In summary, we have successfully developed a general method based on template-assisted ALD to synthesize closely contacted CoO x Pt/TiO 2 and spatially separated CoO x /TiO 2 /Pt catalysts, achieving the precise tuning of CoO x –Pt intimacy by varying the deposition sequence and the wall thickness of the TiO 2 nanotubes. We discover that hydrogen spillover effect generated by the addition of CoO x can cause the increase in O v , providing the adsorption sites for CALD via C=O bond and correspondingly resulting in the enhancement of selectivity to CALC in the CALD hydrogenation reactions. This hydrogen spillover effect is not broken even when we selectively deposit additional oxide layers on the CoO x promoter by ALD to cover its surface entirely. Our work has demonstrated an efficient strategy based on ALD for the design of various bicomponent catalysts with distinct promoter–metal intimacy and the assembly of metals and oxide supports, which is helpful to reveal the origin of bicomponent synergy, the enhancement mechanism and the real active sites. Synthesis of CNCs and the ALD process The detailed CNC synthesis process and the ALD process can be found in our previous reports [24] , [25] , [26] . Synthesis of TiO 2 /Pt catalysts CNCs were firstly decorated with Pt nanoparticles by Pt ALD (20 cycles) and then coated with a TiO 2 layer (300 cycles) by TiO 2 ALD, producing TiO 2 /Pt/CNCs. After the ALD processes, TiO 2 /Pt/CNCs were calcinated at 500 °C for 2 h in air to remove the CNC templates, obtaining TiO 2 /Pt catalysts, in which Pt nanoparticles were confined in TiO 2 nanotubes. Synthesis of CoO x /TiO 2 /Pt catalysts The above-obtained TiO 2 /Pt catalysts were then deposited with cobalt oxides (denoted as CoO x ) by CoO x ALD (150 cycles), obtaining shell-isolated CoO x /TiO 2 /Pt catalysts. Synthesis of CoO x Pt/TiO 2 catalysts CNCs were firstly coated with a TiO 2 amorphous film by TiO 2 ALD, and then Pt nanoparticles were deposited on the TiO 2 /CNCs by Pt ALD obtaining Pt/TiO 2 /CNCs composites. Subsequently, CNCs were removed by calcination under an air atmosphere producing Pt/TiO 2 catalysts with porous anatase nanotubes. Lastly, CoO x nanoparticles were deposited on the outer surface of Pt/TiO 2 through CoO x ALD, producing CoO x Pt/TiO 2 catalysts with the closest CoO x –Pt intimacy. Synthesis of CoO x /TiO 2 /Pt/TiO 2 catalysts CNCs were first coated with a TiO 2 layer (150 cycles) by TiO 2 ALD and then decorated with Pt nanoparticles by Pt ALD and another TiO 2 layer (300 cycles) producing TiO 2 /Pt/TiO 2 /CNCs. After the ALD processes, TiO 2 /Pt/TiO 2 /CNCs were calcinated at 500 °C for 2 h in air to remove the CNC templates, obtaining sandwich-like TiO 2 /Pt/TiO 2 catalysts, in which Pt nanoparticles are coated by the two-layer TiO 2 . Lastly, the obtained TiO 2 /Pt/TiO 2 catalysts were decorated with CoO x nanoparticles by CoO x ALD producing CoO x /TiO 2 /Pt/TiO 2 . Synthesis of Al 2 O 3 /CoO x /TiO 2 /Pt catalysts CNCs were sequentially decorated with Pt nanoparticles by CoO x ALD, coated with a TiO 2 layer (300 cycles) by TiO 2 ALD, decorated with Pt nanoparticles by Pt ALD and then coated with an Al 2 O 3 layer (100 cycles) by Al 2 O 3 ALD producing Al 2 O 3 /CoO x /TiO 2 /Pt/CNCs, which were calcinated at 550 °C for 2 h in air to remove the CNC templates obtaining Al 2 O 3 /CoO x /TiO 2 /Pt catalysts, in which CoO x nanoparticles were covered by the outer Al 2 O 3 layer. Catalyst characterizations TEM and HRTEM images were taken with a JEOL-2100F field-emission transmission electron microscope operated at 200 kV. HAADF-STEM images and EDS mapping profiles were collected on a JEOL ARM-200F field-emission transmission electron microscope operated at 200 kV. The X-ray diffraction (XRD) patterns were recorded by using a Philips X’Pert Pro Super X-ray diffractometer with Cu Kα radiation ( λ = 1.540 Å) in the 2 θ range from 10° to 90°. The X-ray photoelectron spectra (XPS) were collected on an ESCALab-250 X-ray photoelectron spectrometer with an Al Kα source (1486.6 eV). The XANES and EXAFS spectra of the Pt L 3 -edge and Co K-edge were measured on the BL14W1 beamline of the Shanghai Synchrotron Radiation Facility (SSRF), Shanghai Institute of Applied Physics (SINAP), China, operated at 3.5 GeV. A Si (111) double-crystal monochromator was used to reduce the harmonic component of the monochrome beam. Pt foil, PtO 2 , Co foil, CoO and Co 3 O 4 were used as reference samples and measured in the transmission mode, and all the catalysts were also measured in the transmission mode. The diffuse reflectance infrared Fourier transform spectroscopy (DRIFTS, CO chemisorption) measurements were performed on a Bruker Vector 22 spectrometer. After the sample was loaded, it was firstly reduced by 10%H 2 /Ar at 150 °C for 1.5 h. Then the sample was cooled to 30 °C under 10%H 2 /Ar atmosphere, on which a background spectrum was collected. Subsequently, CO was introduced onto the sample until saturation, followed by Ar purge to remove the physically adsorbed gaseous CO. Finally, CO-DRIFTS spectra were collected with 250 scans. H 2 -TPR experiments were performed in a tubular quartz reactor (TP-5080, Tianjin Xianquan, China), into which 50 mg sample was loaded. The reduction was conducted in a 10% H 2 /N 2 atmosphere at a heating rate of 10 °C/min. H 2 -TPD experiments were performed in the same apparatus. A 50-mg sample was firstly reduced in situ at 250 °C for 1 h in a 10% H 2 /N 2 flow and then cooled to 30 °C in the same atmosphere. Subsequently, the sample was swept with nitrogen at a flow rate of 30 sccm for 30 min to remove physisorbed or weakly bound species. TPD was performed by heating the sample from room temperature to 800 °C at a ramp rate of 10 °C/min in nitrogen. N 2 adsorption–desorption experiments were performed on a BELSORP-Mini system at 77 K. The specific surface area was determined using the Brunauer–Emmett–Teller (BET) method, and the pore size distributions were calculated by the Barrett–Joyner–Halenda (BJH) method according to the desorption branches. The Pt and Co metal content of the samples was determined by inductively coupled plasma mass spectrometry (ICP-MS) analysis (Thermo ICAP 6300). Catalytic activity measurements CALD hydrogenation reactions were performed on the above catalysts in a 50-mL stainless-steel autoclave reactor. The reaction was carried out at 65 °C and 2.0 MPa H 2 with a certain amount of catalysts in 30 mL of ethanol, and 100 μL of CALD. After the reaction, the reactor was cooled and then slowly depressurized. Finally, the reaction mixture was separated by centrifugation in order to remove the solid catalysts. The reaction products were analyzed and quantified by gas chromatographic mass spectrometry (GC-MS, Agilent, 7890A). The reaction conversion and selectivity were determined by the product analysis. Computational method Periodic DFT calculations within the generalized gradient approximation (GGA) were conducted with the Vienna ab initio Simulation Package (VASP 5.3.5) with considering the spin-polarization, in which a projector-augmented potential (PAW) method is implemented. The Perdew–Burke–Ernzerhof (PBE) functional at the GGA level was used, and the plane wave basis set was cut off at the energy of 400 eV. For our ALD-prepared cobalt-based catalysts, the obtained cobalt oxides consist of Co 3 O 4 and CoO and the main species is CoO. Therefore, CoO was selected for DFT calculations. The CoO surface was modeled with a six GGA extension atomic layer 3 × 3 CoO(111) slab. DFT + U corrections (an effective onsite Coulomb interaction parameter) were employed to mitigate the self-interaction errors of Co 3d orbital with U-J of 7.1 eV. The main exposed crystal plane for ALD-prepared TiO 2 is the thermodynamically most stable (101) surface, and thus (101) surface was chosen as a model for the anatase TiO 2 interface. The TiO 2 surface was modeled with a six atomic layer 3 × 3 slab. The slab and its image were separated by a vacuum region of 15 Å. The reactant molecular and the top two layers of these model systems were relaxed, whereas other atoms were fixed in their initial lattice sizes.